RecurrentESR1–CCDC170rearrangements in an aggressive subset of oestrogen receptor-positive breast cancers Characterizing the genetic alterations leading to the more aggressive forms of oestrogen receptor-positive (ER+) breast cancers is of critical significance in breast cancer management. Here we identify recurrent rearrangements between the oestrogen receptor gene ESR1 and its neighbour CCDC170, which are enriched in the more aggressive and endocrine-resistant luminal B tumours, through large-scale analyses of breast cancer transcriptome and copy number alterations. Further screening of 200 ER+ breast cancers identifies eight ESR1 – CCDC170 -positive tumours. These fusions encode amino-terminally truncated CCDC170 proteins (ΔCCDC170). When introduced into ER+ breast cancer cells, ΔCCDC170 leads to markedly increased cell motility and anchorage-independent growth, reduced endocrine sensitivity and enhanced xenograft tumour formation. Mechanistic studies suggest that ΔCCDC170 engages Gab1 signalosome to potentiate growth factor signalling and enhance cell motility. Together, this study identifies neoplastic ESR1 – CCDC170 fusions in a more aggressive subset of ER+ breast cancer, which suggests a new concept of ER pathobiology in breast cancer. The crucial role of recurrent gene fusions in the development of solid tumours has been recently appreciated after several milestone discoveries [1] , [2] . In particular, the discovery of an EML4 – ALK fusion in ~4% of lung cancer has led to the development of an effective drug with stunning clinical impacts [3] . Recently, next-generation sequencing has greatly enhanced gene fusion discovery in solid tumours, which has led to the identification of a VTI1A – TCF7L2 fusion in 3% of colon cancers [4] , a BCOR – CCNB3 fusion in 4% of bone sarcomas [5] and a FGFR – TACC fusion in 3% of glioblastomas [6] . Although low in percentage, these neoplastic gene fusions will likely advance the genetic subtyping of solid tumours that may be curable by targeting them. In breast cancer, a recent RNA sequencing (RNAseq) study reported multiple fusions of the MAST and NOTCH family genes, whereas individual gene fusions appear to rarely recur [7] . Another genome sequencing study revealed a MAGI3 – AKT3 gene fusion in 3% of breast cancers that is enriched in triple-negative tumours [8] . To date, the role of recurrent fusions in oestrogen receptor-positive (ER+) breast cancers is ill understood. ER + breast cancers can be classified into the ‘luminal A’ and ‘luminal B’ subtypes. Although luminal A tumours can be effectively treated by endocrine therapy against the ER, the luminal B subtype tumours are more aggressive with a higher risk of early relapse with endocrine therapy [9] . It has been unclear what drives these tumours to be more aggressive, and there are limited options for treating this type of cancer. These issues may be effectively addressed by uncovering the genetic aberrations that drive the development of these tumours. In this study, we develop an integrative pipeline called ‘Fusion Zoom’ to detect recurrent gene fusions from RNAseq and genomic data sets. We postulate that the detection of pathological gene fusions would be greatly improved by applying more sensitive parameters to comprehensively capture the authentic fusion sequences from the RNAseq data, and by integrating distinct types of genomic data to prioritize the driving fusion events. Based on the observation that gene rearrangements are frequently associated with intragenic copy number aberrations (or ‘unbalanced’ breakpoints), we previously formulated a fusion breakpoint principle to describe the characteristic intragenic copy number changes delineating recurrent fusion genes [10] , which empowers the bioinformatics analysis to catalogue meaningful fusion genes from copy number data. To facilitate high-throughput biological interpretation of candidate fusions, we also developed a Concept Signature (ConSig) analysis that nominates biologically important genes underlying cancer by assessing their association with molecular concepts characteristic of cancer genes [10] ( http://consig.cagenome.org ). Based on these principles, here we develop a pipeline that detects recurrent chimeras potentially encoding in-frame protein products from RNAseq data, catalogues the unbalanced breakpoints at the genomic loci of these fusion partner genes from copy number data and prioritizes pathological gene fusions through the ConSig analysis ( Fig. 1a , see Methods). We apply this approach to the RNAseq and copy number data sets from The Cancer Genome Atlas (TCGA), and identify neoplastic fusion events between the oestrogen receptor gene ESR1 and the adjacent gene CCDC170 in a subset of ER+ breast cancers that is preferentially found in luminal B tumours. 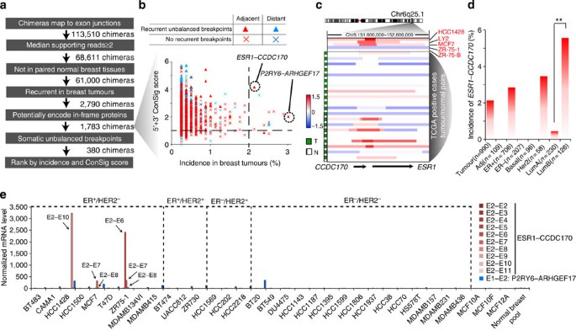Figure 1: Discovering recurrent gene fusions in invasive breast cancer. (a) The workflow of the Fusion Zoom pipeline. (b) Prioritizing fusion candidates by copy number breakpoints, ConSig score and incidence in breast cancer. (c) Log2 transformed copy number data at theCCDC170/ESR1locus forESR1–CCDC170-positive cell lines and tumours (LY2 and ZR-75-B are derivative clones of MCF7 and ZR-75-1, respectively). T, tumour, N, normal blood from the same patient (in three cases, paired normal breast tissues are shown as blood tissues are not available). Copy number data for index breast cancer cell lines and tumours are from Heiseret al.44and TCGA49, respectively. (d) The incidence ofESR1–CCDC170fusion in different breast cancer clinical subtypes. **P<0.01 (Fisher’s exact test). (e) Nanostring analysis of 30 breast cancer cell lines reveals the presence ofESR1–CCDC170in HCC1428, ZR-75-1 and MCF7 cells. E2–E2, E2–E3… E2–E11: exon 2 ofESR1is fused to exons 2, 3 …11 ofCCDC170. The exon numbers are based on reference sequence NM_001122742 forESR1, NM_025059 forCCDC170, NM_176796 forP2RY6, and NM_014786 forARHGEF17. Figure 1: Discovering recurrent gene fusions in invasive breast cancer. ( a ) The workflow of the Fusion Zoom pipeline. ( b ) Prioritizing fusion candidates by copy number breakpoints, ConSig score and incidence in breast cancer. ( c ) Log2 transformed copy number data at the CCDC170 / ESR1 locus for ESR1 – CCDC170- positive cell lines and tumours (LY2 and ZR-75-B are derivative clones of MCF7 and ZR-75-1, respectively). T, tumour, N, normal blood from the same patient (in three cases, paired normal breast tissues are shown as blood tissues are not available). Copy number data for index breast cancer cell lines and tumours are from Heiser et al. [44] and TCGA [49] , respectively. ( d ) The incidence of ESR1 – CCDC170 fusion in different breast cancer clinical subtypes. ** P <0.01 (Fisher’s exact test). ( e ) Nanostring analysis of 30 breast cancer cell lines reveals the presence of ESR1 – CCDC170 in HCC1428, ZR-75-1 and MCF7 cells. E2–E2, E2–E3… E2–E11: exon 2 of ESR1 is fused to exons 2, 3 …11 of CCDC170 . The exon numbers are based on reference sequence NM_001122742 for ESR1 , NM_025059 for CCDC170 , NM_176796 for P2RY6 , and NM_014786 for ARHGEF17 . Full size image Integrative analysis revealed a recurrent ESR1 rearrangement Using the Fusion Zoom pipeline, we analysed the RNAseq data of 795 invasive breast tumours and 107 paired normal breast tissues from TCGA. A total of 113,510 putative gene fusions were detected, among which 2,790 fusions were found to be tumour-specific and recurrent in this cohort of patients (present in ≥2 tumours). Among these recurrent fusion candidates, 1,783 are found to have the potential to encode in-frame protein products (see Methods). Interestingly, the vast majority of these recurrent chimeras were from genes that are less than 500 kb apart ( Fig. 1b ), whereas distant gene fusions rarely recurred in more than 1% of breast tumours ( Fig. 1b ). Chimeras from adjacent genes are generally considered as non-genomic transcription-induced chimeras (TIC) resulting from intergenic splicing [11] , [12] . Interestingly our analysis of TCGA copy number data (SNP6.0) for 865 breast tumours (most of these tumours have matched RNAseq data) did reveal somatic unbalanced breakpoints within a subset of tumours expressing chimeras, suggesting that some of these fusions could be the consequence of DNA rearrangements. To further reveal the most frequent and pathologically relevant fusions, we classified the 1,783 fusion candidates based on the presence of recurrent unbalanced breakpoints (see Methods), and then prioritized these candidates based on their frequency of detection in breast tumours and by ConSig score of fusion genes ( Fig. 1b ). This analysis nominated two lead candidates, ESR1 – CCDC170 and P2RY6–ARHGEF17, among which ESR1 – CCDC170 is most frequently associated with unbalanced breakpoints among all candidates expressed in >1% of breast tumours ( Fig. 1c ). Next, we examined the expression of both candidates in a panel of 30 breast cancer cell lines by Nanostring analysis, which applies nanoparticles to detect the abundance of target transcripts from total RNA [13] . This assay detected high levels of ESR1 – CCDC170 expression in some but not all of these cell lines ( Fig. 1e ). The three ESR1 – CCDC170 -positive cell lines, MCF7, ZR-75-1 and HCC1428, are all ER+ and derived from metastatic breast tumours. The sizes of the fusion variants detected in these cell lines are different, suggesting that different genomic regions are involved in the fusion events ( Fig. 1e and Supplementary Fig. 1a ). In addition, none of the benign breast epithelial cell lines or pooled normal breast tissues harbours the ESR1 – CCDC170 fusion. These data suggest that ESR1 – CCDC170 may be an authentic recurrent gene fusion. P2RY6–ARHGEF17 was expressed at a modest level in many of the breast cancer cell lines analysed ( Fig. 1e and Supplementary Fig. 1b ). We speculated that this is most likely a TIC and thus did not study it further. ESR1 – CCDC170 is expressed in more aggressive ER+ tumours ESR1 encodes the oestrogen receptor, whereas CCDC170 encodes a protein with unknown function. CCDC170 is broadly expressed at modest levels in human tissues, with the fallopian tube to be the highest expressing organ ( Supplementary Fig. 2 ). In normal breast tissues, CCDC170 is expressed at a moderate level. To date, there is no report about the role of CCDC170 in mammary gland biology. The observed fusions between ESR1 and CCDC170 join the 5′-untranslated region of ESR1 upstream to the coding region of CCDC170 , enabling the expression of truncated CCDC170 under the promoter of the ESR1 gene. To more accurately capture the ESR1 – CCDC170 chimerical reads from RNAseq data, we reconstructed all possible variant sequences by randomly combining each of the exons of ESR1 with that of CCDC170 . Aligning these putative sequences with the RNAseq data for 990 tumours (released to date by TCGA) revealed 21 ESR1 – CCDC170- positive breast tumours (all of which are ER+, except one indeterminate case). About 55% of these positive tumours showed copy number gains between the ESR1 and CCDC170 loci as shown in Fig. 1c (also see Supplementary Table 1 ). Analysis of clinicopathological data [14] suggests that this fusion is preferentially present in the luminal B rather than the luminal A subtype (Fisher’s exact test, P <0.01, see Fig. 1d ). In contrast, wild-type (wt) CCDC170 is broadly expressed in ER+ breast tumours, with no significant difference between these two luminal subtypes ( Supplementary Fig. 3 ). The expression of wt CCDC170 in breast cancer cell lines is almost exclusive to ER+ lines ( Supplementary Fig. 1a ). This is consistent with the previous report about its co-expression with ESR1 [15] . We then tested the presence of ESR1 – CCDC170 in 200 ER+ breast tumours by reverse transcription PCR (RT–PCR), using primers from exon 2 of ESR1 and exon 10 of CCDC170 , which can detect most fusion variations. Among these tumours, eight showed strong expression of ESR1 – CCDC170 (4%), which were verified by capillary sequencing ( Fig. 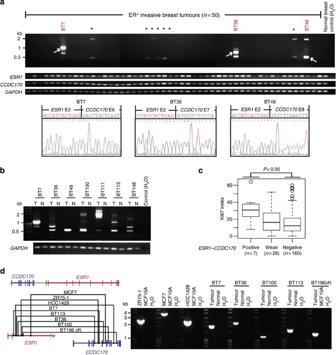Figure 2: Characterization of theESR1–CCDC170fusion in breast cancer cell lines and tissues. (a) Representative RT–PCR results ofESR1–CCDC170, wtESR1and wtCCDC170in ER+ breast cancer tissues. Asterisk (*) represents weakESR1–CCDC170transcripts detected by RT–PCR. (b) RT–PCR analysis ofESR1–CCDC170in paired tumour (T) and adjacent normal tissues (N) from seven strong positive cases. (c) The Ki67 index forESR1–CCDC170positive, weak and negative cases evaluated by IHC assay using available tissue sections for 193 ER+ cases assessed forESR1–CCDC170expression.P-value was determined byt-test. (d) Genomic PCR analysis of the positive cell lines and five strong positive tumour samples, confirming theESR1–CCDC170rearrangements. Left panel shows the schematic of identified genomic fusion points in different samples; right panel shows the gel image ofESR1–CCDC170genomic PCR products. Hash (#) indicates paired normal tissue is not available for BT196. 2a and Supplementary Table 2 ). In contrast, no expression of these fusion variants was detected in the available paired adjacent normal breast tissues, suggesting that the fusion between ESR1 and CCDC170 is highly tumour-specific ( Fig. 2b ). Figure 2: Characterization of the ESR1 – CCDC170 fusion in breast cancer cell lines and tissues. ( a ) Representative RT–PCR results of ESR1 – CCDC170 , wt ESR1 and wt CCDC170 in ER+ breast cancer tissues. Asterisk (*) represents weak ESR1 – CCDC170 transcripts detected by RT–PCR. ( b ) RT–PCR analysis of ESR1 – CCDC170 in paired tumour (T) and adjacent normal tissues (N) from seven strong positive cases. ( c ) The Ki67 index for ESR1–CCDC170 positive, weak and negative cases evaluated by IHC assay using available tissue sections for 193 ER+ cases assessed for ESR1 – CCDC170 expression. P -value was determined by t -test. ( d ) Genomic PCR analysis of the positive cell lines and five strong positive tumour samples, confirming the ESR1 – CCDC170 rearrangements. Left panel shows the schematic of identified genomic fusion points in different samples; right panel shows the gel image of ESR1 – CCDC170 genomic PCR products. Hash ( # ) indicates paired normal tissue is not available for BT196. Full size image To examine the association of ESR1 – CCDC170 with the luminal B subtype, we assayed Ki67 expression by immunohistochemistry (IHC) in the ER+ cases assessed by RT–PCR for ESR1 – CCDC170 . Ki67 is a proliferation biomarker, and a high Ki67 index has been used in the clinic to classify luminal B tumours (with a cutoff of 13–15% positivity) [16] , [17] , [18] . Among the 200 ER+ cases, 193 cases had evaluable tissue sections for Ki67 IHC analysis. The IHC results showed that ESR1 – CCDC170 -positive cases have significantly higher Ki67 scores than negative cases ( Fig. 2c , Supplementary Fig. 4 ). Using 15% positivity as cutoff, 80 tumours have high Ki67 index, among which 6 cases are fusion positive (7.5%); among the 113 Ki67-low tumours, only one tumour is fusion positive (0.9%). Fisher’s exact test suggests a significant enrichment of fusion-positive cases in Ki67-high tumours ( P =0.02). This data support the association of ESR1 – CCDC170 with the more aggressive luminal B subtype. ESR1 – CCDC170 genomic rearrangements and protein products ESR1 and CCDC170 are located 69 kb apart on chromosome 6 with CCDC170 positioned 5′ of ESR1 . This placement prevents strong cis -splicing events that frequently happen between neighbouring genes placed in forward order. 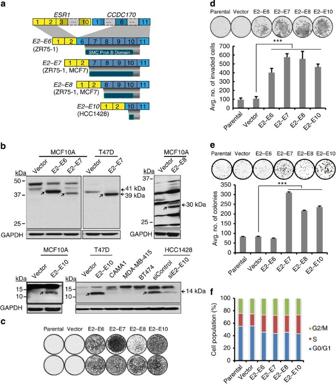Figure 3: Characterization ofESR1–CCDC170 protein products and their transforming activity in MCF10A breast epithelial cells. (a) Schematic ofESR1–CCDC170fusion variants and encoded proteins identified in breast cancer cell lines. ORFs are depicted in dark shades. The exon numbers are based on reference sequence NM_001122742 forESR1and NM_025059 forCCDC170. (b) Immunoblot analysis of MCF10A and T47D cells expressing ΔCCDC170 ORFs, the fusion-positive HCC1428 cell line and fusion-negative control cell lines, using an anti-CCDC170 polyclonal antibody. Arrows indicate the ΔCCDC170 bands. To enhance the detection of differentially sized ΔCCDC170 protein variants, the blot region pertaining to the molecular weight of each respective ΔCCDC170 variant was cut and then probed with the antibody. A longer exposure time is required to enhance the visualization of the E2–E8 fusion protein. The identity of the 14 kDa band detected in HCC1428 is verified by an siRNA against the E2–E10 fusion expressed by this line. Overexpression of ΔCCDC170 variants in MCF10A cells significantly enhances (c) cell migration, (d) matrigel invasion and (e) clonal expansion. (f) Cell cycle analysis of the MCF10A cell models. Error bars represent the s.d. of at least three replicate measurements per condition. The results shown are representative of experiments performed at least twice. ***P<0.001 (t-test). ‘Vector’ indicates MCF10A cells transduced with pLenti7.3 vector containing an YFP ORF. To further verify the genomic origin of ESR1 – CCDC170 in the cell lines and tumours showing strong expression of the chimeras, we carried out genomic PCR using tiling primers designed for the specific ESR1 or CCDC170 intron regions suspected to harbour the rearrangement based on the fusion variant in each index case revealed by RT–PCR ( Supplementary Table 3 ), and the amplified products were further analysed by capillary sequencing. Using this approach, the genomic fusion points in all three fusion-positive cell lines and five out of eight strong fusion-positive tumours have been successfully identified ( Fig. 2d ). The sequencing results revealed distinct genomic fusion points in different cell lines and tumours. The MCF7 cells showed a duplication of the fusion junction, whereas the remaining cases showed 1–10 base pair homology between the ESR1 and CCDC170 sequences at the rearrangement junctions ( Supplementary Fig. 5 ). We then examined the structure of the four major fusion variants (E2–E6, E2–E7, E2–E8 and E2–E10) detected in both breast cancer cell lines and tumours, in which exon 2 of ESR1 is fused to exon 6, 7, 8 or 10 of CCDC170 . The common theme of these fusion variants appears to create different-sized amino-terminally truncated CCDC170 proteins (ΔCCDC170), while ESR1 does not contribute to any of the fusion amino-acid sequence ( Fig. 3a ). To identify the protein products of the four major fusion variants, we ectopically expressed the putative open reading frames (ORFs) of these variants in MCF10A human breast epithelial cells ( Supplementary Fig. 6a ). Western blot analysis using a commercial polyclonal antibody against the carboxy terminus of CCDC170 detected the predicted 41 kDa (E2–E6), 39 kDa (E2–E7), 30 kDa (E2–E8) or 14 kDa (E2–E10) ΔCCDC170 bands specific to the transduced MCF10A cells ( Fig. 3b ). In addition, we expressed the E2–E7 and E2–E10 ORFs in the fusion-negative T47D breast cancer cells (ER+), and detected proteins of the same sizes. Next, we performed western blot analysis to detect the endogenously expressed ΔCCDC170 proteins in the ESR1 – CCDC170 -positive cell lines. We were able to readily detect the 14 kDa E2–E10 protein expressed by the HCC1428 cells, the identity of which has been verified by specific knockdown of the E2–E10 fusion using an small interfering RNA against this fusion junction ( Fig. 3b ). We were unable to conclusively detect the endogenous proteins expressed by the ZR-75-1 or MCF7 cell lines presumably because of the presence of cross-reactive proteins or low expression levels, respectively ( Supplementary Fig. 7 ). Figure 3: Characterization of ESR1 –CCDC170 protein products and their transforming activity in MCF10A breast epithelial cells. ( a ) Schematic of ESR1 – CCDC170 fusion variants and encoded proteins identified in breast cancer cell lines. ORFs are depicted in dark shades. The exon numbers are based on reference sequence NM_001122742 for ESR1 and NM_025059 for CCDC170 . ( b ) Immunoblot analysis of MCF10A and T47D cells expressing ΔCCDC170 ORFs, the fusion-positive HCC1428 cell line and fusion-negative control cell lines, using an anti-CCDC170 polyclonal antibody. Arrows indicate the ΔCCDC170 bands. To enhance the detection of differentially sized ΔCCDC170 protein variants, the blot region pertaining to the molecular weight of each respective ΔCCDC170 variant was cut and then probed with the antibody. A longer exposure time is required to enhance the visualization of the E2–E8 fusion protein. The identity of the 14 kDa band detected in HCC1428 is verified by an siRNA against the E2–E10 fusion expressed by this line. Overexpression of ΔCCDC170 variants in MCF10A cells significantly enhances ( c ) cell migration, ( d ) matrigel invasion and ( e ) clonal expansion. ( f ) Cell cycle analysis of the MCF10A cell models. Error bars represent the s.d. of at least three replicate measurements per condition. The results shown are representative of experiments performed at least twice. *** P <0.001 ( t -test). ‘Vector’ indicates MCF10A cells transduced with pLenti7.3 vector containing an YFP ORF. Full size image ESR1 – CCDC170 endows more aggressive phenotypes Next, we sought to examine the oncogenic potential of the ΔCCDC170 proteins generated by the four ESR1 – CCDC170 fusion variants in the MCF10A breast epithelial cells. Impressively, ectopically expressing the ORF of each of these fusion variants dramatically increased the migration and invasion capabilities as shown by the Boyden chamber assay ( Fig. 3c,d ). In addition, the E2–E7 and E2–E10 variants also induced a moderate but significant increase in cell proliferation and colony-forming ability, as measured by MTT assay ( Supplementary Fig. 6b ) and clonogenic assay ( Fig. 3e ), respectively. Soft agar colony formation assays did not show an increase in anchorage-independent growth of the engineered MCF10A cells, whereas three-dimensional culture of these cells in Matrigel revealed impaired acini morphogenesis ( Supplementary Fig. 6c ). Cell cycle analysis revealed an increase in S-G2/M phase cells, and a decrease in G0/G1 phase cells in all models ( Fig. 3f ). As MCF10A cells do not express wt CCDC170 (see Supplementary Fig. 1a ), the observed changes are likely to be independent of wt CCDC170 . To investigate the role of ESR1 – CCDC170 in ER+ breast cancer cells, we examined the phenotypic changes of T47D breast cancer cells ectopically expressing the E2–E7 or E2–E10 fusions or the wt CCDC170 (as a control). T47D is a luminal breast cancer cell line that is highly dependent on oestrogen [19] . Our data show that while both E2–E7 and E2–E10 fusions significantly increased cell motility, anchorage-independent growth and colony-forming ability of T47D cells, the wt CCDC170 did not ( Fig. 4a–c ). Further, both the E2–E7 and E2–E10 variants rendered the T47D cells less sensitive to oestrogen deprivation and 4-hydroxytamoxifen treatment (the active metabolite of tamoxifen used in vitro ) ( Fig. 4d,e ). Of note, T47D cells typically do not proliferate when deprived of oestrogen, whereas ΔCCDC170 transduced T47D cells continue to grow in the absence of oestrogen and irrespective of tamoxifen treatment ( Fig. 4d ). Moreover, ΔCCDC170 enhanced the ER transcriptional activity in the presence of oestrogen but not with endocrine therapy ( Supplementary Fig. 8a ), suggesting that the fusion-mediated endocrine-sensitivity changes are unlikely due to the restoration of ER activity. To further examine the oncogenic potential of ΔCCDC170 in the in vivo context, we transplanted the T47D cells expressing the ΔCCDC170 variants or vector control into female athymic nude mice implanted with estradiol (E2) pellets. Impressively, in contrast to the slow growth kinetics of the tumour in the vector control group, a profound increase in tumour growth was observed in the transduced xenograft models expressing E2–E7 or E2–E10 ORFs ( Fig. 4f and Supplementary Fig. 8b ). In addition, immunostaining of tumour tissue arrays revealed that T47D xenograft tumours overexpressing ΔCCDC170 variants have a Ki67 index significantly greater than that of control T47D tumours ( Fig. 4g ). 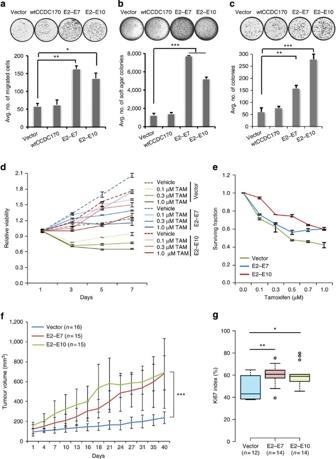Figure 4:ESR1–CCDC170endows more aggressive phenotypes in T47D ER+ breast cancer cells. Ectopic expression of ΔCCDC170 in T47D cells results in a significant increase in (a) cell motility, (b) anchorage-independent growth and (c) colony-forming ability. (d) Time-point changes in the proliferation of fusion-expressing T47D cells after tamoxifen treatment (4-OHT). (e) Surviving fraction of T47D cells expressing ΔCCDC170 after 7 days of 4-OHT. In assayd,e, T47D cells are deprived of oestrogen for tamoxifen treatment. Error bars represent the standard deviation of two replicate measurements per condition and results shown are representative of experiments performed at least twice. (f) The growth curve of xenograft tumours expressing vector, E2–E7 or E2–E10 ΔCCDC170 variants engrafted bilaterally in athymic nude mice (8 mice per group). Tumour volumes of deceased mice are not included after the day of death. Day 1 represents the first tumour measurement 7 days post tumour cell implantation. Data are presented as mean±s.d. of indicated sample size. (g) Boxplots comparing the Ki67 scores in available xenograft tumour tissues expressing vector (n=12), E2–E7 (n=14) or E2–E10 (n=14). ‘Vector’ indicates the pLenti7.3 vector control containing an YFP ORF. *P<0.05, **P<0.01, ***P<0.001 (theP-value forFig. 4fis based on analysis of variance, and others are all based ont-test). Figure 4: ESR1 – CCDC170 endows more aggressive phenotypes in T47D ER+ breast cancer cells. Ectopic expression of ΔCCDC170 in T47D cells results in a significant increase in ( a ) cell motility, ( b ) anchorage-independent growth and ( c ) colony-forming ability. ( d ) Time-point changes in the proliferation of fusion-expressing T47D cells after tamoxifen treatment (4-OHT). ( e ) Surviving fraction of T47D cells expressing ΔCCDC170 after 7 days of 4-OHT. In assay d , e , T47D cells are deprived of oestrogen for tamoxifen treatment. Error bars represent the standard deviation of two replicate measurements per condition and results shown are representative of experiments performed at least twice. ( f ) The growth curve of xenograft tumours expressing vector, E2–E7 or E2–E10 ΔCCDC170 variants engrafted bilaterally in athymic nude mice (8 mice per group). Tumour volumes of deceased mice are not included after the day of death. Day 1 represents the first tumour measurement 7 days post tumour cell implantation. Data are presented as mean±s.d. of indicated sample size. ( g ) Boxplots comparing the Ki67 scores in available xenograft tumour tissues expressing vector ( n =12), E2–E7 ( n =14) or E2–E10 ( n =14). ‘Vector’ indicates the pLenti7.3 vector control containing an YFP ORF. * P <0.05, ** P <0.01, *** P <0.001 (the P -value for Fig. 4f is based on analysis of variance, and others are all based on t -test). Full size image To further investigate the function of endogenous ESR1 – CCDC170 , we examined the consequence of specific knockdown of this fusion in HCC1428 cells harbouring the E2–E10 variant. This cell line was chosen for the knockdown model as the E2–E10 variant is amenable to the design of fusion-specific siRNA and is the only variant expressed by this cell line. In addition, the protein product of this variant is readily detectable by the available antibody, which can be used to examine the knockdown efficiency. As shown in Fig. 3b and Supplementary Fig. 9 , this siRNA effectively and specifically knocks down the E2–E10 fusion variant. MTT and Boyden chamber assays revealed that repression of the E2–E10 fusion by siRNA in HCC1428 cells potently inhibited their growth and diminished their migration towards the fibroblast attractant, while no significant effect was observed in the fusion-negative MDA-MB-415 cells ( Fig. 5a,b ). To further exclude the siRNA off-target effects in HCC1428 cells, we performed rescue experiments by ectopically expressing the E2–E10 fusion variant in this line. Forced expression of E2–E10 variant rescued the knockdown effect of E2–E10 siRNA on proliferation of HCC1428 cells ( Supplementary Fig. 10 ). This result further corroborated the role of the endogenous E2–E10 fusion expressed in HCC1428 cells. 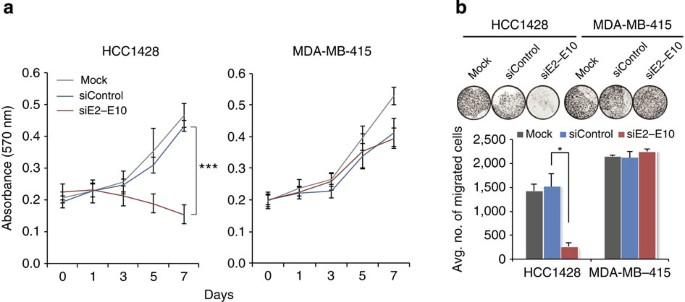Figure 5: Evaluating the function of the endogenousESR1–CCDC170fusion in HCC1428 breast cancer cells by genetic inhibition. (a) Knockdown ofESR1–CCDC170in HCC1428 cells impairs cell proliferation (MTT assay). Error bars represent the s.d. of four replicate measurements per condition. ***P<0.001 (t-test based on day 7 data). (b) Knockdown ofESR1–CCDC170in HCC1428 cells impairs cell motility as revealed by transwell migration assay. NIH 3T3 cells are used as chemo attractant. The fusion-negative MDA-MB-415 cell line (ER+/Her2−) was used as negative control. Error bars represent the s.d. of two replicate measurements per condition. The results shown are representative of experiments performed at least twice. *P<0.05 (t-test). Figure 5: Evaluating the function of the endogenous ESR1 – CCDC170 fusion in HCC1428 breast cancer cells by genetic inhibition. ( a ) Knockdown of ESR1 – CCDC170 in HCC1428 cells impairs cell proliferation (MTT assay). Error bars represent the s.d. of four replicate measurements per condition. *** P <0.001 ( t -test based on day 7 data). ( b ) Knockdown of ESR1 – CCDC170 in HCC1428 cells impairs cell motility as revealed by transwell migration assay. NIH 3T3 cells are used as chemo attractant. The fusion-negative MDA-MB-415 cell line (ER+/Her2−) was used as negative control. Error bars represent the s.d. of two replicate measurements per condition. The results shown are representative of experiments performed at least twice. * P <0.05 ( t -test). Full size image ESR1 – CCDC170 engages Gab1 signalosome To investigate the key oncogenic pathways that characterize the ESR1 – CCDC170- positive tumours, we performed gene set enrichment analyses (GSEA) using the matched Agilent gene profiling data from TCGA to select differentially expressed genes between fusion-positive and negative tumours. Among the top upregulated pathways in ESR1 – CCDC170 -positive tumours, the signalling gene sets along the c-Met/Gab1/PI3K-AKT axis appear to be most relevant to the observed phenotypes ( Supplementary Fig. 11a ). Of particular interest is the upregulation of the Gab1 signalosome ( Fig. 6a ). Gab1 is a key docking protein that enhances the downstream signalling of c-Met and many other receptor tyrosine kinases [20] , [21] , and is also a key scaffold protein involved in the formation of invadopodia [22] . Further analysis revealed significant upregulation of Gab1 but not c-Met in the fusion-positive breast tumours ( Supplementary Fig. 11b ). Interestingly, when ΔCCDC170 variants were overexpressed in MCF10A or T47D cells, Gab1 was also upregulated; conversely, repression of ΔCCDC170 reduced Gab1 protein level in HCC1428 cells ( Fig. 6b ). In contrast, c-Met protein levels were not increased in the MCF10A and T47D cells expressing ΔCCDC170, and were not affected by E2–E10 knockdown in HCC1428 cells. 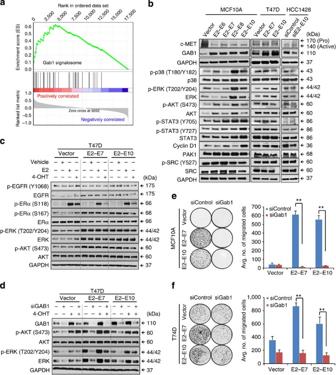Figure 6:ESR1–CCDC170may engage Gab1 to enhance cell motility and augment growth factor signalling. (a) The representative enrichment plot of upregulated Gab1 signalosome genes inESR1–CCDC170-positive breast tumours versus the same number of randomly selected luminal B tumours. Please seeSupplementary Fig. 11afor more details of this analysis. (b) Western blot showing the alterations of signalling molecules in MCF10A or T47D cells overexpressing ΔCCDC170 variants, or following knockdown of the E2–E10 fusion in HCC1428 cells. (c) The impact of ΔCCDC170 expression on ERα, EGFR, AKT and ERK levels and phosphorylations in T47D cells in the context of serum starvation and endocrine treatment. Cells were deprived of oestrogen and serum, and then treated with vehicle, 1 nM oestrogen (E2) or 100 nM 4-hydroxy tamoxifen (4-OHT) for 20 min. (d) Alterations of AKT and ERK activities following GAB1 knockdown in transduced T47D cells. Cells were deprived of oestrogen, transfected with GAB1 siRNA for 72 h and treated with 100 nM 4-OHT for 20 min.e,f, The impact of Gab1 knockdown on fusion-driven cell motility in MCF10A (e) and T47D (f) cells. Error bars represent the s.d. of two replicate measurements per condition. The results shown are representative of experiments performed at least twice. **P<0.01 (t-test). Figure 6: ESR1 – CCDC170 may engage Gab1 to enhance cell motility and augment growth factor signalling. ( a ) The representative enrichment plot of upregulated Gab1 signalosome genes in ESR1 – CCDC170 -positive breast tumours versus the same number of randomly selected luminal B tumours. Please see Supplementary Fig. 11a for more details of this analysis. ( b ) Western blot showing the alterations of signalling molecules in MCF10A or T47D cells overexpressing ΔCCDC170 variants, or following knockdown of the E2–E10 fusion in HCC1428 cells. ( c ) The impact of ΔCCDC170 expression on ERα, EGFR, AKT and ERK levels and phosphorylations in T47D cells in the context of serum starvation and endocrine treatment. Cells were deprived of oestrogen and serum, and then treated with vehicle, 1 nM oestrogen (E2) or 100 nM 4-hydroxy tamoxifen (4-OHT) for 20 min. ( d ) Alterations of AKT and ERK activities following GAB1 knockdown in transduced T47D cells. Cells were deprived of oestrogen, transfected with GAB1 siRNA for 72 h and treated with 100 nM 4-OHT for 20 min. e , f , The impact of Gab1 knockdown on fusion-driven cell motility in MCF10A ( e ) and T47D ( f ) cells. Error bars represent the s.d. of two replicate measurements per condition. The results shown are representative of experiments performed at least twice. ** P <0.01 ( t -test). Full size image Next, we performed western blot analysis to examine the impact of ΔCCDC170 expression on Gab1 downstream signalling molecules ( Supplementary Fig. 11c ). This revealed the positive correlation of phospho AKT, ERK, and p38 with ΔCCDC170 expression, the extent of which varies between different models ( Fig. 6b ). To test if ΔCCDC170 expression can result in hyperactive growth factor signalling irrespective of endocrine condition, the T47D cell models were deprived of oestrogen for 48 h and serum-starved for 24 h, and then treated with vehicle, E2 or tamoxifen. Interestingly, sustained phosphorylation of AKT and ERK was observed in the T47D cells expressing ΔCCDC170 even after withdrawal of oestrogen and serum, and this effect was not significantly altered by the administration of oestrogen or tamoxifen ( Fig. 6c ). This suggests that the hyperactive growth factor signalling observed with ΔCCDC170 expression may not be attributed to the oestrogen-regulated non-genomic ER activity known to modulate growth factor signalling [23] . Further, increased phosphorylation of the Serine 167 residue on ERα was observed with ΔCCDC170 expression. This site has been reported to be phosphorylated by both AKT and ERK, enhancing ERα transcriptional activity [24] . Gab1 silencing using a documented siRNA [25] counteracted the enhanced AKT and ERK signalling driven by ΔCCDC170 ( Fig. 6d , Supplementary Fig. 11d ), suggesting that ESR1 – CCDC170 may act through Gab1 to augment growth factor signalling. Of note, Gab1 repression cannot diminish AKT activation in the presence of tamoxifen, suggesting that tamoxifen may bypass Gab1 and engage some other mechanism to activate AKT, possibly through tamoxifen-activated non-genomic ER activity [26] . Further, Gab1 knockdown also diminished the fusion-driven cell motility in both MCF10A and T47D cells, supporting the importance of Gab1 signalling in the fusion-driven invasive programme ( Fig. 6e,f ). The genetic makeup and underlying biology contributing to the highly proliferative and aggressive phenotype of the luminal B breast tumours is not well understood. In this study, we have identified a recurrent genomic rearrangement event between the ESR1 and CCDC170 loci, and provided strong molecular and functional evidence that this fusion is enriched in luminal B tumours and promotes more aggressive oncogenic phenotypes. Our finding of ESR1 – CCDC170 is an example of gain-of-function mutation, wherein CCDC170 is fused to ESR1 and utilizes the constitutively active promoter of ER to drive the expression of a truncated form of CCDC170 gene. The truncation of the CCDC170 protein resulting from this fusion may twist the biology of this protein and generate a phenotype distinct from the wild-type protein. Of note, ESR1 – CCDC170 is also detected by two previous studies interrogating different RNAseq data sets as a candidate fusion in breast cancer which further support its recurrence [7] , [27] . However, these studies did not provide any data on the genomic event underlying this fusion, or its pathobiology and clinical relevance in breast cancer. Our integrative bioinformatics analysis provided multiple clues to lock in on this fusion as a recurrent, pathological, genomic fusion event from the large number of putative fusions detected by RNAseq. We then validated the genomic rearrangements generating this fusion by genomic PCR, characterized its protein products, elucidated its pathological role and engaged mechanism, and verified its enrichment in the more aggressive luminal B subtype. While it remains to be answered whether such enrichment could be attributable to the increased genomic instability characteristic of luminal B tumours that may promote the formation of this fusion, our biological data show that ESR1 – CCDC170 endows ER+ breast cancer cells with more aggressive phenotypes, such as enhanced cell migration, invasion, anchorage-independent growth and reduced endocrine sensitivity. These properties are consistent with the behaviour of luminal B tumours. In addition, we also observed markedly increased Ki67, the luminal B marker, in the T47D xenograft tumours overexpressing ΔCCDC170 variants. Moreover, our ‘knockdown/rescue’ studies of the E2–E10 fusion expressed in the HCC1428 cell line, which encodes the smallest truncated version of CCDC170 that is retained in all fusion variants, provided a proof of concept for the function of the endogenous ESR1 – CCDC170 fusions expressed in breast cancers. Further mechanistic studies suggest that this fusion may engage Gab1 signalling to enhance cell motility and augment the downstream signalling of growth factor receptors [28] . More important, the enhancement of growth factor signalling driven by this fusion appears to be sustained even after withdrawal of serum, and is not affected by endocrine treatment. Together, these findings may shed light on the genetic aberrations underlying the more aggressive and fatal ER+ breast tumours. Our RT–PCR analysis of ER+ breast tumour tissues revealed 8 out of 200 tumours as ESR1 – CCDC170 -positive cases with strong expression of this fusion (4%). Of note, besides these cases, we also observed weak expression of ESR1 – CCDC170 in an additional 10% of ER+ breast tumours, which are distinguishable from the strong positives (see methods). These weak cases show a slightly increased Ki67 index comparing to fusion-negative breast tumours but this difference is not statistically significant ( Fig. 2c ). We speculate that these may be the result of random weak trans -splicing events between ESR1 and CCDC170, considering the vicinity of the two genes. In fact, such trans -splicing events are not unique to this fusion [29] . Oncogenic gene fusions resulting from distant translocations are often found to be expressed at a low level in normal tissues, such as the EML4–ALK [30] , NPM–ALK [31] , JAZF1–JJAZ1 (ref. 32 ) and BCR–ABL1 fusions [33] . It is thought that high-level expressions coincide with gene rearrangements, whereas low-level expressions are likely to be trans -splicing events [32] . Nevertheless, we cannot exclude the possibility of ESR1 – CCDC170 rearrangements in a small subset of cancer cells in rare cases. Thus further investigation is needed to elucidate their clinical significance. Another interesting question about this fusion is how such cryptic rearrangements could be generated. As CCDC170 is located to the 5′ of ESR1 on the same DNA strand, it is unlikely that such rearrangements are generated by deletions or inversions, which would require CCDC170 to be at the 3′ of ESR1 , or on the opposite strand, respectively. Considering the frequent duplications between the two genes in fusion-positive tumours, one possible mechanism of these cryptic rearrangements could be tandem duplication, which is defined as the occurrence of two identical sequences, one following the other, in a chromosome segment. Tandem duplication has been found to cause other gene fusions in cancer [34] , [35] , [36] . If this mechanism is responsible for ESR1 – CCDC170 fusions, ESR1 expression would not be disrupted as such rearrangements are likely to retain a copy of the wt ESR1 while forming the fusion gene ( Supplementary Fig. 12a ), as reported for other gene fusions generated by tandem duplication [37] . Indeed, the expression of ESR1 in ESR1 – CCDC170 -positive tumours is similar to that of fusion-negative ER+ breast tumours ( Supplementary Fig. 12b ). In addition to tandem duplication, more complex mechanisms such as insertions may be responsible in the positive cases that do not exhibit duplications between the ESR1 and CCDC170 loci ( Fig. 1c ). Chimeras from adjacent genes account for a vast majority of chimera sequences in cancer transcriptome [38] , [39] . Our finding of the ESR1 – CCDC170 gene fusions supports the possibility of chromosomal rearrangements between adjacent genes generating recurrent gene fusions. Such cryptic genetic changes are not generally detectable by conventional cytogenetic approaches, and the resulting chimeras are usually submerged in the overwhelming number of transcription-induced chimeras [38] , [39] . This finding suggests that special attention should be paid to the possible genomic origin of adjacent chimeras in the discovery of gene fusions from RNAseq data. To our knowledge, ESR1 – CCDC170 could be the most important recurrent gene fusion yet reported in ER+ breast cancers. This discovery may shed new light on the special genetic aberrations underlying a subset of more aggressive ER+ breast cancers, and offers a new diagnostic strategy to identify this group of patients for more appropriate treatments. Further studies are needed to comprehensively investigate the oncogenic process initiated by the ΔCCDC170 proteins resulting from this fusion and elucidate their role in breast cancer endocrine resistance. Analyses of RNAseq and copy number data The copy number and RNAseq (Illumina HiSeq, paired-end) data for breast tumours used in this study were from TCGA ( http://cancergenome.nih.gov/ and https://cghub.ucsc.edu ). Paired-end RNA sequences for 795 breast tumours and 107 paired normal breast tumours were aligned to human genome build 19 using the Tophat 2.0 fusion junction mapper [40] . Using our Perl script pipeline called ‘Fusion Zoom’, the putative fusion junctions were mapped to human exons (derived from UCSC gene and Ensemble gene) to identify chimerical sequences. The putative gene fusions are required to be supported by a minimum of one read that maps to the exon junctions of the two fusion genes. This criterion was expected to filter out most artifactual gene fusions randomly ligated during the sequencing procedure. This is based on the fact that authentic gene fusion junctions are usually formed by exon boundaries of partnering genes, whereas the fusion junctions of these artifactual fusions are unlikely to coincide with exon boundaries [41] . Putative fusion sequences were then constructed and aligned against human genome and transcriptome using the accurate aligner BLAST. The chimeric sequences that can mostly align to a wt genomic or transcript sequence were disregarded. After such filtering, a total of 68,611 chimeras with >2 median number of reads across all tumours were identified. A total of 2,790 putative fusions were identified as somatic and recurrent (present in more than one breast tumours). Among these, 1,783 putative fusions were found to have the potential to encode in-frame protein products. Here the in-frame analysis detects a fusion that either results in an in-frame chimerical protein, or combines the untranslated 5′ UTR of the 5′ partner with the full-length ORF of the 3′ partner. This is computed based on the reading frames of the respective UCSC and Ensemble wt transcripts. The ORF analysis based on the reading frames of exons of the partner genes cannot predict all the de novo ORFs generated by the fusions. Here we required the candidate fusion to present an in-frame fusion variant in at least one sample. This step filtered out about 1,000 candidates that never present any in-frame variant in any single sample, which are less likely to be functionally relevant. Of note, this approach cannot detect a truncated ORF initiated by an internal ATG site (such as in ESR1 – CCDC170 fusions). However, in rare cases, the TCGA-positive tumour appears to express the ESR1 – CCDC170 variant that involves more 5′ exons of ESR1 , thus generating a reading frame with a small fragment of ESR1 ORF in-frame fused to truncated CCDC170 ORF. This triggers the programme to consider this fusion as potentially encoding in-frame ORF. The fusion candidates were then ranked by the incidence of fusion transcripts in breast tumours and the ConSig score ( http://consig.cagenome.org , release 2) [10] . To assess the unbalanced breakpoints within candidate fusion genes, we obtained TCGA ‘level 3’ Affymetrix SNP6.0 copy number data for 865 breast tumours. These level 3 data are generated by circular binary segmentation [42] . The genomic position of each copy number transition was mapped with the genomic regions of all human genes. The genomic region of each human gene was designated as the starting of the transcript variant most approaching the 5′ of the gene, and the end of the variant most approaching the 3′ of the gene. The ‘broken’ genes with intragenic copy number breakpoints were classified into candidate 5′ and 3′ partners based on the association of these unbalanced breakpoints with gene placements. The 5′ amplified genes or 3′ deleted genes were considered as potential 5′ partners, while 5′ deleted or 3′ amplified genes were considered as potential 3′ partners according to the fusion breakpoint principle [10] . The copy number transitions within the ESR1/CCDC170 loci were manually assessed using segmented copy number data visualized with integrative genomics viewer [43] ( Fig. 1c ). Copy number data for index breast cancer cell lines are from Heiser et al. [44] Fusion-associated copy number gain is defined as increased copy number in-between CCDC170 and ESR1 loci comparing with 5′ CCDC170 and 3′ ESR 1 regions (visually assessed based on segmented copy number data at ESR1/CCDC170 loci). Thus copy number gain also includes the case where both 5′ CCDC170 and 3′ ESR1 regions have copy number loss. The 380 recurrent fusion candidates revealed by the above integrative analysis are provided in Supplementary Data 1 . Please refer to http://fusionzoom.cagenome.org for more details of the pipeline. To more accurately capture ESR1 – CCDC170 chimerical reads, we reconstructed all putative fusion-variant transcripts by combining each of ESR1 exons with each of the CCDC170 exons. The resulting putative ESR1 – CCDC170 variant sequences are provided in Supplementary Data 2 . Using the Burrows–Wheeler Aligner, we aligned these ESR1 – CCDC170 variant sequences with the RNAseq data for 990 breast tumours released to date by TCGA, allowing up to three mismatches. Using a Perl script, we processed the Bam output files to identify junction or encompassing chimerical reads. A series of filtering steps were performed to remove the false positives due to misalignments. The raw sequences of fusion reads identified after these filtering are provided in Supplementary Data 3 . A breast tumour was considered as fusion-positive if Burrows–Wheeler Aligner revealed a minimum of three chimerical reads with at least one read mapped to the fusion junction. To assure that the alignments are acceptable, paired reads supporting ESR1 – CCDC170 were manually realigned with the respective putative variant sequences as well as the human transcriptome and genome reference sequences using BLAST or BLAT. For index tumours with <10 supporting fusion reads, all fusion reads were curated. For index tumours with ≥10 supporting fusion reads, all junction reads and at least 10 fusion mates (if available) were curated. The curation results are provided in Supplementary Data 3 . PAM50-based clinical subtypes of breast cancer for TCGA samples were derived from the TCGA publication [45] . The clinical data for TCGA samples were obtained from UCSC Cancer Genome Browser [46] . Gene expression data analysis Gene set enrichment analysis (GSEA) was done by comparing the ESR1 – CCDC170 -positive breast tumours profiled by gene expression array (data from TCGA), with the same number of randomly chosen fusion-negative luminal B breast tumours, using a signal-to-noise ratio algorithm. The curated canonical pathways from the Molecular Signatures Database ( http://www.broadinstitute.org/gsea/msigdb/ ) were used as the gene set database. The process of randomly selecting fusion-negative luminal B samples and then performing GSEA analyses was repeated 100 times. The normalized enrichment scores for each pathway were averaged and then ranked to identify consensus-enriched pathways ( Supplementary Fig. 11a ). Gene expression data for normal human tissues (Affymetrix U133 plus 2.0) are from the human body index data set (GSE7307), and are analysed using Oncomine ( www.oncomine.org ). Cell line and tissue collections Breast cancer cell lines were obtained from American Type Culture Collection including the NCI-ATTC ICBP 43 cell line kit. All breast tumour tissues were obtained from the Tumor Bank of the Lester and Sue Smith Breast Center at Baylor College of Medicine. The total RNA for normal breast tissues (5 Donor Pool) was purchased from BioChain (R1234086-P). Nanostring assay The code sets for the ESR1 – CCDC170 and P2RY6–ARHGEF17 fusion variants were designed by Nanostring Technologies based on the fusion junction sequences. Expressions of these fusion variants were quantified from 500 ng total RNAs using the Nanostring nCounter Assay System following the manufacturer’s instructions. Raw counts were normalized to the messenger RNA levels of the house-keeping genes TFRC , TBP and PUM1 . RT–PCR and genomic PCR Complementary DNA was generated from 1 μg of total RNA using the Transcriptor First Strand cDNA Synthesis Kit (Roche) in the presence of both oligo (dT) and random primers. RT–PCR of the ESR1 – CCDC170 fusion was performed with Platinum Taq High Fidelity (Invitrogen) and fusion-specific primers (Forward: 5′-CTGCGGTACCAAATATCAGCAC-3′; Reverse: 5′-CTTCTCCAGTTGGTCTCTGGAT-3′). To avoid contamination, a clean room was used for setting up PCR reactions, which is separated from the areas used for thermal cycling and manipulation of PCR products. In addition, a special set of pipettes and tips with aerosol filters was used to set up the PCR reaction. All cDNA samples were subjected to 35 PCR cycles of 94 °C for 30 s, 56 °C for 30 s and 68 °C for 2 min. For semi-quantification of RT–PCR results, band intensities were quantified using ImageJ software (National Institutes of Health) and normalized to respective GAPDH controls. A relative value more than 0.8 was considered as positive for ESR1 – CCDC170 fusion. All the weak cases had a relative value below 0.3. Genomic PCR was carried out with 200–300 ng of genomic DNA from cell lines or tissues using the Expand Long Range PCR system (Roche) and primers listed in Supplementary Table 3 . PCR products were gel purified for capillary sequencing (Lone Star Labs or Beckman Coulter Genomics). The ESR1 – CCDC170 genomic fusion sequences revealed by capillary sequencing are provided in Supplementary Data 4 . Ki67 IHC Formalin-fixed paraffin-embedded (FFPE) whole tissue sections (for breast cancer tissues) or tissue microarrays (20 tissue cores/slide) (for T47D xenograft tumours) were stained using a mouse Ki67 monoclonal antibody (MIB1 clone, Dako) as previously described [47] . Briefly, microwave-assisted heat-induced retrieval for antigen epitopes was performed in Tris–HCl buffer, at pH 9.0 for 10 min. Endogenous peroxidase activity was blocked by incubation in a 3% hydrogen peroxide for 10 min. The primary antibody MIB1 at dilution of 1:200 was incubated for 1 h at room temperature, followed by incubations with polymer labelled EnVision+ HRP reagents (DAKO, #K4001) and DAB substrate (DAKO, #K3468). The slides were then counterstained with Harris’ hematoxylin. Normal human tonsil was used as positive control. Immunostaining was evaluated by two pathologists who were blinded to the sample information, according to recommendations from the international Ki67 working group [48] . Briefly, the section was first scanned at low magnification (10–20 × ) to determine the most representative areas. The Ki67 index was calculated as the percentage of Ki67-positive cells among a total of 500 cells at 40 × magnification. For heterogeneous cases with hot spots, the Ki67 index was calculated as the average percentage of Ki67-positive cells among a total of 250 cells in hot spots and 250 cells in other areas. In vitro overexpression of ESR1 – CCDC170 ORFs The cDNA fragments of E2–E6, E2–E7, E2–E8 or E2–E10 fusion variants containing the full-length ORFs were amplified from ZR-75-1 or HCC1428 cDNAs using Phusion DNA polymerase (NEB) with the forward primer 5′-CCATGCTCCTTTCTCCTGCCCA-3′ from 5′ ESR1 , and reverse primer 5′-TGTGCCATGTCTTATGGCCACCT-3′ from the 3′ untranslated region of CCDC170 . The predicted ORFs of these four variants and YFP control were then cloned into the pLenti7.3 vector (Invitrogen). The ORF sequences of ESR1 – CCDC170 fusion variants are provided in Supplementary Data 5 . After verification by sequencing, these lentiviral constructs were infected into selected cell lines using the ViraPower Lentiviral Support Kit (Invitrogen). Cells with high GFP reporter expression were selected using flow cytometry. siRNA knockdown experiments The E2–E10-specific siRNA (5′-CAUCACUGAGAUUAAAACU-3′) and Gab1-specific siRNA (siGenome GAB1: 5′-GAGAGUGGAUUAUGUUGUU-3′) were purchased from Dharmacon. All siRNAs were transfected using Lipofectamine RNAi MAX Reagent (Invitrogen) according to manufacturer’s instructions. Western blot Protein samples were separated in SDS–PAGE gel and transferred either onto 0.2 μm polyvinylidene fluoride membrane for detection of the E2–E10 protein product, or 0.2 μm nitrocellulose membrane for other proteins. The dilutions of primary antibodies used were 1:250–1:1,000 for rabbit anti-CCDC170 (GeneTex), 1:1,000 for mouse anti-c-Met and rabbit anti-Gab1 (Cell Signaling) and other antibodies. Antibodies were obtained from Santa Cruz (cyclin D1), Thermo Fisher (ERα), Abcam (PAK1), Millipore (Src) and Cell Signaling (all other molecules). To study the fusion-driven signalling in the condition of serum withdrawal and endocrine treatment, cells were maintained in phenol red-free medium for 48 h, serum-starved for 24 h and then treated for 20 min with vehicle (Ethanol), 17β-estradiol (E2) (1 nM) or Tam (100 nM). 4-OH tamoxifen (Tam) and 17β-estradiol (E2) were obtained from Sigma-Aldrich. Cell proliferation assay Cell proliferation was measured by MTT assay using the Cell Proliferation kit I (Roche) according to manufacturer’s instructions. For tamoxifen sensitivity studies, cells were oestrogen deprived (ED) for 48 h using phenol red-free medium with charcoal-dextran-stripped fetal bovine serum, seeded (1,000–2,500 cells per well) in 96-well plates, and exposed to varying doses of Tam (0.1–1.0 μM); cell proliferation was assessed after 7 days. The surviving fraction of cells was calculated by dividing the OD value from drug-treated wells by the OD value of vehicle-treated wells. Clonogenic assay Cells were seeded at a density of 300–500 cells per well in 6-well plate and incubated for 14–21 days. As ΔCCDC170 promotes the formation of large-sized colonies, the colonies>350 μm in diameter were counted for comparison, using GelCount (Oxford Optronix). Soft agar colony formation assay Cells were suspended in growth medium containing 0.35% SeaPlaque Agarose (Lonza), and plated at a density of 5,000 cells per well in a 6-well plate containing 0.7% base agar in growth medium. The cells were then incubated for 14 days, and colonies ≥100 μm in diameter were counted using GelCount. Migration and invasion assay Transwell migration and invasion assays were performed using Boyden chambers. Cells were serum starved for 24 h and seeded at a density of 5 × 10 4 –2 × 10 5 in serum-free medium onto transwell inserts of 8 μm pore size for migration assay, or onto transwell chambers coated with Matrigel (BD Biosciences) for invasion assay. To facilitate the migration of HCC1428 and MDA-MB-415 cells, NIH3T3 cells seeded in the bottom chamber served as chemoattractant. After 48–72 h, the inserts were fixed in 4% formaldehyde and stained with hematoxylin and eosin. ERE luciferase reporter assay Cells were co-transfected with 1 μg of an ERE (oestrogen transcriptional response element) luciferase reporter construct (ERE-TK-Luc) and 0.1 μg of pCMV β-galactosidase as an internal control for transfection efficiency in serum-free medium using XtremeGene HP (Roche). The luciferase levels were measured with a Luciferase Reporter Assay kit (Promega) in a luminometer and normalized to β-gal activity. Fluorescence-activated cell sorting analysis For cell cycle analysis, propidium iodide-stained cells were analysed in a LSRFortessa cell analyzer (BD Biosciences), and cell cycle phases were calculated using FlowJo ( www.flowjo.com ). In vivo xenograft experiments All animal work has been approved by the BCM Institutional Animal Care and Use Committee. A quantity of 2 × 10 7 transduced T47D cells were resuspended in 20% Matrigel solution, and were transplanted bilaterally to 4–6-week old female athymic nude mice supplemented with 60-day-release 17β-estradiol pellets. Xenograft tumours of the T47D models were successfully engrafted in eight mice per group. The growth of the xenograft tumours was monitored twice per week and tumour volume was measured using the formula 1/2(length × width 2 ). Statistical analysis For the in vivo study, statistical comparison of tumour volumes was performed using one-way analysis of variance. The results of all in vitro experiments were analysed by Student’s t -tests, and all data are shown as mean±s.d. How to cite this article : Veeraraghavan, J. et al. Recurrent ESR1 – CCDC170 rearrangements in an aggressive subset of oestrogen receptor-positive breast cancers. Nat. Commun. 5:4577 doi: 10.1038/ncomms5577 (2014).